Quantum teleportation from a propagating photon to a solid-state spin qubit A quantum interface between a propagating photon used to transmit quantum information and a long-lived qubit used for storage is of central interest in quantum information science. A method for implementing such an interface between dissimilar qubits is quantum teleportation. Here we experimentally demonstrate transfer of quantum information carried by a photon to a semiconductor spin using quantum teleportation. In our experiment, a single photon in a superposition state is generated using resonant excitation of a neutral dot. To teleport this photonic qubit, we generate an entangled spin–photon state in a second dot located 5 m away and interfere the photons from the two dots in a Hong-Ou-Mandel set-up. Thanks to an unprecedented degree of photon-indistinguishability, a coincidence detection at the output of the interferometer heralds successful teleportation, which we verify by measuring the resulting spin state after prolonging its coherence time by optical spin-echo. Quantum teleportation [1] has attracted considerable interest not only as a versatile quantum-state-transfer method but also as a quantum computational primitive [2] , [3] , [4] . Over the last decade, both probabilistic/heralded [1] , [5] , [6] , [7] , [8] and deterministic teleportation [9] , [10] , [11] , [12] , [13] have been demonstrated in various quantum systems. The realization of quantum teleportation between a propagating photon and a single semiconductor spin that we describe in this paper closely builds on prior demonstrations of photon—stationary qubit interfaces in collective atomic excitations in atomic vapours [14] , [15] and in doped crystals [16] , [17] , as well as in single trapped atoms [18] , [19] . Semiconductor quantum dots (QDs) have been at the forefront of two seemingly uncorrelated approaches to experimental quantum information science [20] : on the one hand, single QDs in photonic nanostructures have been used to realize high-efficiency sources for single photons [21] , [22] , [23] , [24] with potential applications in quantum key distribution [25] and linear optics quantum computation [3] . On the other hand, single spins confined in QDs have been extensively studied as promising solid-state qubits with long coherence time and a potential for integration on a chip [26] , [27] , [28] , [29] , [30] , [31] . By realizing teleportation of the quantum state of a photonic qubit generated by one QD to the spin state of another QD located in a different cryostat, we demonstrate that these two auspicious features of QDs can be combined to realize an elementary process relevant for a quantum network [32] , [33] . In our experiments, the photonic qubit is a near-transform-limited single photon pulse prepared in a superposition of two frequency (colour) components, which we label as ω b and ω r . The frequency spread around each component, primarily determined by the inverse pulse-width, is much smaller than ω b – ω r . A photonic/frequency qubit with these basic properties is naturally generated upon fast resonant excitation of a neutral QD where the properties of the excitation laser uniquely determining the quantum state of the generated single photon pulse in an optical mode A. The target spin confined in a single-electron-charged QD is prepared in a maximally entangled state [34] , [35] , [36] with a second photonic frequency qubit propagating in a second, distinct mode B. The key step in photon-to-spin quantum teleportation protocol we implement is the two-photon interference of the photons in modes A and B in a Hong-Ou-Mandel (HOM) interferometer [1] . Provided that the input photonic modes are indistinguishable in all aspects except for their internal qubit state, detection of a coincidence event at the output of the HOM interferometer heralds the successful completion of teleportation: if the photonic qubit in mode A was initially prepared in | ψ p >= α | ω b › A + β | ω r › A , the output QD electron spin state will be | ψ e >= α |↓›+ β |↑›. Here, |↑› (|↓›) denotes electron spin parallel (anti-parallel) to the external magnetic field direction. The experiments described in this paper entail several major advances necessary for the demonstration of heralded quantum teleportation. A crucial element in this endeavour is the assurance of the indistinguishability of the two photonic qubits. To attain this goal, we use resonant laser excitation as well as local electric and magnetic field control of the transition energies of the QDs, yielding an unprecedented degree of two-photon interference visibility of 82±2%. Given the propagation time delays, it is also essential that the QD spin remains coherent for about 10 ns needed to complete the teleportation protocol. QD electron spins on the other hand, have a relatively short dephasing time (~1 ns) determined by the effective random, but quasi-static, magnetic field stemming from hyperfine interactions with the QD nuclei. To ensure that the spin–photon entanglement remains intact during the time needed to herald teleportation, we have implemented an all-optical spin-echo sequence and prolonged the lifetime of spin–photon entanglement from 1 to 13 ns. Finally, verification of successful teleportation of four different photonic qubit states is achieved by carrying out single electron spin measurements conditioned on a coincidence detection at the output of the HOM interferometer. Indistinguishable photonic frequency qubits In a neutral self-assembled InGaAs QD, the elementary optical excitations from the unique ground state |0› are the two fundamental exciton states X r and X b that are split in energy by the anisotropic electron-hole exchange interaction. In our experiments, the photonic qubit to be teleported is generated by resonant-pulsed excitation of these excitonic transitions. The exciton state X r ( X b ) decays at rate Γ 1 by spontaneous emission of a photon at frequency ω r ( ω b ) back into |0›. A laser pulse resonant with either of these two exciton states results in the generation of a single-colour single photon states denoted by | ω b ›, | ω r ›. Alternatively, applying a two-colour laser pulse that is simultaneously resonant with both X r and X b results in the superposition state α | ω b ›+ β | ω r ›. The left-hand side of Fig. 1 shows the experimental set-up we use to generate such a single-photon state. The two-colour laser pulse that excites the QD is obtained by tuning the frequency of a diode laser exactly in the middle of the two neutral exciton transitions and sending the beam to an amplitude electro-optic modulator (EOM) that generates 800 ps pulses (for the two-photon interference experiment in Fig. 2 ) or 400 ps pulses (for the teleportation experiment) from the continuous-wave laser field. A phase EOM (Ph-EOM) is used to generate laser sidebands that are on resonance with the exciton transitions, and enable us to resonantly drive X r and X b simultaneously. The amplitude of the modulation signal is set such that the central (carrier) peak at the laser frequency is completely suppressed. In this way, most of the laser power is carried by the frequencies ω b and ω r . Two orthogonal polarizers on the excitation and collection paths of the QD, set at | H + V › and | H − V ›, respectively, are used to suppress the laser background. The complex, time-varying electric field of the modulated laser pulse, after passing the excitation polarizer, at the location of the QD has the form , where Δ= ω b – ω r and φ L is the tunable relative phase imprinted by phase modulation. E H + V ( t ) denotes the amplitude-modulated complex electric field emitted by the laser. The synchronization scheme (Methods and Supplementary Fig. S1 ) ensures that φ L has the same constant value for each repetition of the experiment. 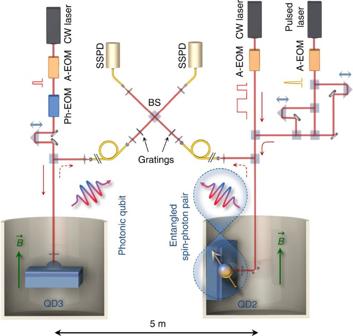Figure 1: Experimental set-up. The neutral exciton transitions in a single InGaAs QD (QD3) are resonantly excited by a 0.4 ns laser pulse. Upon spontaneous emission the QD generates a photon in an experimentally tunable superposition state of the two neutral exciton transition frequencies, forming a single photon qubit. A different QD (QD2) in the single-electron charged state, under a perpendicular external magnetic field, is resonantly excited by a sequence of pulses that initialize the electron spin and excite the blue negatively charged exciton (trion). An entangled spin–photon pair is generated upon spontaneous emission from the trion state. The two QDs are located in separate liquid helium bath cryostats that are ~5 m apart. The emitted single photons from the two QDs are collected into single mode fibres and sent to interfere on a beam splitter in a Hong-Ou-Mandel set-up. In both arms, transmission gratings with 70 GHz bandwidth are used to filter out the 200 GHz detuned 4 ps rotation laser as well as the phonon sideband emission from the QDs. SSPDs are used to detect the photons on the output arms of the beam splitter. A coincidence detection on the two SSPDs heralds a successful teleportation of the state of the photonic qubit to that of the electron spin in QD2, which is measured by the same two SSPDs at a later time. Figure 1: Experimental set-up. The neutral exciton transitions in a single InGaAs QD (QD3) are resonantly excited by a 0.4 ns laser pulse. Upon spontaneous emission the QD generates a photon in an experimentally tunable superposition state of the two neutral exciton transition frequencies, forming a single photon qubit. A different QD (QD2) in the single-electron charged state, under a perpendicular external magnetic field, is resonantly excited by a sequence of pulses that initialize the electron spin and excite the blue negatively charged exciton (trion). An entangled spin–photon pair is generated upon spontaneous emission from the trion state. The two QDs are located in separate liquid helium bath cryostats that are ~5 m apart. The emitted single photons from the two QDs are collected into single mode fibres and sent to interfere on a beam splitter in a Hong-Ou-Mandel set-up. In both arms, transmission gratings with 70 GHz bandwidth are used to filter out the 200 GHz detuned 4 ps rotation laser as well as the phonon sideband emission from the QDs. SSPDs are used to detect the photons on the output arms of the beam splitter. A coincidence detection on the two SSPDs heralds a successful teleportation of the state of the photonic qubit to that of the electron spin in QD2, which is measured by the same two SSPDs at a later time. 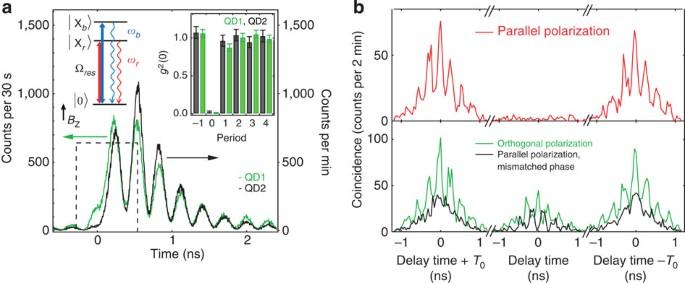Figure 2: Photon indistinguishability of two frequency photonic qubits. (a) Time resolved resonance fluorescence counts are plotted for QD1 (green) and QD2 (black). A 0.8 ns two colour laser pulse (dashed line) that is resonant with both excitonic transitions |Xb› and |Xr› excites the QD (left inset); subsequent spontaneous emission generates a single photon in a superposition ofωbandωr. The matched oscillations of the emission from the two QDs at Δ=ωb–ωr=3.45 GHz indicate that the generated photonic qubit states are nearly identical. The right inset shows photon correlation (g2) measurements on the two QDs using the emitted photons detected after the excitation pulse is turned off, indicating that the likelihood of two or more photon detection events is very small. The error bars represent 1 s.d., deduced from poissonian statistics of the raw detection events. (b) The photonic qubits depicted inaare incident on a beam splitter. Coincidence counts on the two output arms of the beam splitter are plotted as a function of the delay between the recorded photon arrival times.T0is the pulse repetition time of 13.1 ns. As the photons are indistinguishable when the input modes have parallel polarization (top panel), the coincidence counts within the time window (−1.2 ns, 1.2 ns) are 11 times smaller than those in which the second photon is detected in other periods. In the bottom panel, the photons are rendered distinguishable either through their polarization (green) or their phase (black), leading to a centre peak coincidence count that is two times smaller than the other periods. Full size image Figure 2: Photon indistinguishability of two frequency photonic qubits. ( a ) Time resolved resonance fluorescence counts are plotted for QD1 (green) and QD2 (black). A 0.8 ns two colour laser pulse (dashed line) that is resonant with both excitonic transitions | X b › and | X r › excites the QD (left inset); subsequent spontaneous emission generates a single photon in a superposition of ω b and ω r . The matched oscillations of the emission from the two QDs at Δ= ω b – ω r =3.45 GHz indicate that the generated photonic qubit states are nearly identical. The right inset shows photon correlation ( g 2 ) measurements on the two QDs using the emitted photons detected after the excitation pulse is turned off, indicating that the likelihood of two or more photon detection events is very small. The error bars represent 1 s.d., deduced from poissonian statistics of the raw detection events. ( b ) The photonic qubits depicted in a are incident on a beam splitter. Coincidence counts on the two output arms of the beam splitter are plotted as a function of the delay between the recorded photon arrival times. T 0 is the pulse repetition time of 13.1 ns. As the photons are indistinguishable when the input modes have parallel polarization (top panel), the coincidence counts within the time window (−1.2 ns, 1.2 ns) are 11 times smaller than those in which the second photon is detected in other periods. In the bottom panel, the photons are rendered distinguishable either through their polarization (green) or their phase (black), leading to a centre peak coincidence count that is two times smaller than the other periods. Full size image We assume that the leading edge of the two-colour laser pulse reaches the QD location at time t =0. The state vector of the QD prior to the spontaneous emission event at time t em is then given by , where we assume that | X b › and | X r › are linearly polarized along H and V , respectively. The probability amplitudes a ( t ) and b ( t ) are determined by the laser coupling strength and the spontaneous emission rate. Upon emission at t em the generated photon is in the state , which after the polarizer on the collection path becomes ; as both colour components after the polarizer are polarized along H − V , we drop the polarization index. In the presence of a magnetic field, the | X b › and | X r › transitions are no longer linearly polarized; however, this alters neither the relative phase nor the amplitude of the two colour components of the H − V -polarized photon transmitted by the polarizer. The detection of the photonic frequency qubit can be implemented with a detector having time jitter smaller than 1/Δ. Upon absorption of a photon, the qubit is projected onto the state ; the probability that a photon is registered is then |‹ ψ M | ψ P ›| 2 =[1+cos(2 φ L +Δ t em )]/2. With φ L and Δ fixed, the counts show an oscillation as a function of the photon emission time t em , which can be deduced from the corresponding photon detection time t d . The result is a temporal beat signal stemming from an interference of the two partial waves of the frequency qubit on the single-photon detector. The measurement of a photonic frequency qubit is depicted in Fig. 2a and in Supplementary Fig. S2 : the beats of ω b and ω r demonstrate that the single photon is in a coherent superposition of two frequencies. The finite visibility of the interference of the two frequency components stems predominantly from the jitter of the detector; the excitation pulse jitter also has a non-zero contribution. As indistinguishability of photonic qubits is essential for a high teleportation fidelity, we carried out a two-photon interference experiment using two photonic frequency qubits generated by two QDs (QD1 and QD2) placed in separate cryostats. To ensure good spectral overlap of the emission from the two QDs, we pick one QD and find a second QD in a different cryostat that matches the first QD in photoluminescence (PL) emission wavelength within ±0.03 nm (±10 GHz). For this purpose, we use piezo-scanners to step through a range of our sample which has a density of 0.25 per μm 2 , generating a spatial map of PL emission wavelength for each QD. In this experiment, given the wavelength distribution of our QDs, the probability for one dot to be close to our target PL emission wavelength of 957.5 nm is 1/1,300, implying that a scanning range of ~70 × 70 μm 2 is needed to find a matching QD. Once a pair of QDs with nearly identical PL emission wavelengths is found, the local gate voltages applied separately to the two QDs, yielding a tuning range of ~20 GHz, are used to fine tune their transition frequencies into resonance. To ensure that both ω r and ω b of the two QDs are identical, we additionally apply local magnetic fields. Figure 2b shows the time-resolved coincidences between the two output ports of the HOM interferometer as a function of the time delay between the photon detection times, when the two input photons have either identical or orthogonal polarizations. Our measurements reveal that the visibility is , when we consider the photon emission after the laser pulse in the time window [0.8 ns, 2 ns]. Here, C ⊥ ( C || ) is the total counts in the central peak with orthogonal (parallel) polarization for the input modes of the beam splitter. When the two input photons are in different periods or if they have orthogonal polarizations, then two-photon interference is absent: the observed beat signal in those cases originate exclusively from single-photon interference. We remark that the indistinguishability is further improved when we interfere single-frequency photon pulses: the visibility V =0.82±0.02 we obtain in this case (see Supplementary Fig. S5 ) constitutes a drastic improvement over the previous experiments [37] , [38] . With a retro-reflecting prism in one of the arms of interferometer, we introduce a half-period time delay ( t = π /Δ) for one of the pulses, which also renders the two photonic qubits distinguishable ( Fig. 2b ). For any given arrival time at the beam splitter, such a delay ensures that the relative phase between the two frequency components of the two single photons differs by π . The observed beat notes around the centre period near zero delay time, stem from an interference between the two frequency qubits and ; a similar beat note would be observed for input photons in | ω b › and | ω r › (ref. 39 ). The suppression of the beat signal in different periods in this case stems from a superposition of two π -phase-shifted single-photon interference patterns. The degradation of the interference visibility is discussed in Supplementary Note 1 . Spin–photon entanglement with echo sequence An entangled spin–photon pair can be generated using resonant optical excitation of a single-electron charged QD [34] , [35] , [36] , where the ground states are identified by the orientation of the electron spin. Spontaneous emission of H ( V )-polarized photon at frequency ω r ( ω b ) from the trion state | T r › at rate Γ 2 /2 brings the QD back into the |↓› (|↑›) state, resulting in the maximally entangled state [34] After erasing the polarization information using a polarizer transmitting H − iV polarized light, the spin–photon entangled state reads (ref. 34 ). Here, we indicated that the photon that is entangled with the spin is channelled into the photonic mode B, which constitutes the second input mode of the HOM interferometer ( Fig. 1 ). The entangled state is effected by decoherence of the QD spin. Owing to the hyperfine interaction between the electron spin and QD nuclear spin ensemble, the electron spin is subject to an effective magnetic field determined by a combination of the fixed externally applied field and the quasi-static random Overhauser field. For different repetitions of the experiment the nuclear spins will be in different states, yielding a corresponding slowly fluctuating Overhauser field and thereby decreasing of the timescale that electron spin coherence is observable. This timescale is commonly referred to as spin dephasing time; for our QDs ns. To ensure that the electron spin coherence is intact for a longer time period, we introduce what is referred to as an optical spin-echo sequence [40] that removes the effect of static, but random, Overhauser field (see Supplementary Note 3 for more information about the echo sequence and its effect on decoherence). The electron spin is still subject to decoherence but now at a timescale that is commonly referred to as spin-echo T 2 coherence time . To demonstrate that quantum correlations between the spin and the photon can be prolonged by spin-echo, we start by increasing the applied gate voltage to the QD2 in order to deterministically charge it with a single excess electron. 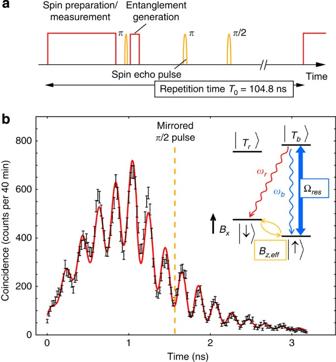Figure 3: Characterization of spin–photon entanglement. (a) The laser pulse sequence used for the generation of spin–photon entangled state and measurement of quantum correlations after a spin-echo sequence. (b) Spin–photon entanglement in the rotated basis and the relevant energy-level diagram (right inset). QD2 is prepared in the single-electron charged state and an external magnetic field ofBx=0.7Tis applied in the Voigt geometry. The main figure shows the photon detection events as a function of time, during and after the entanglement generation pulse, conditioned upon a spin-echo-delayed spin measurement in thestate. The entanglement generation pulse is turned on at timet=0 and is 1.2 ns long. The oscillations in the depicted coincidence counts at Δ=ωb–ωr=4.9 GHz are due to the beating between the two frequency components of the projected single-photon superposition state. The vertical dashed line indicates the entangled spin–photon generation time, for which the spin-echo sequence exactly cancels the random phase accumulated due to hyperfine interactions. The error bars represent 1 s.d., deduced from poissonian statistics of the raw detection events. Figure 3a shows the laser pulse sequence for generating spin–photon entanglement with spin-echo. The relevant energy-level diagram as well as the allowed optical transitions for QD2 under an external magnetic field B x =0.7T that is applied perpendicular to the growth direction (Voigt geometry) are depicted in Fig. 3b (inset). We prepare the QD in |↓› state by applying a 10 ns long resonant laser pulse tuned to the |↑›–| T b › transition. A subsequent 4 ps-long π -pulse transfers the spin onto |↑› (ref. 30 ). This pulse drives a coherent two-photon stimulated Raman transition between the two spin levels and its power is chosen such that it coherently swaps the populations in the states; we refer to such coherent spin manipulation pulses as rotation pulses. An entangled spin–photon pair is then generated by resonant excitation of the | T b › with a 1.2 ns resonant laser pulse which we refer to as the entanglement pulse. The combination of a π -pulse applied at time T echo /2 and a π /2-pulse applied at time T echo implements the spin-echo sequence. The whole pulse sequence is repeated after 104.8 ns, with the subsequent 10-ns long resonant laser implementing spin measurement for the preceding pulse sequence, as well as ensuring spin pumping/preparation in the |↓› state for the next cycle. We discuss measurements of the spin in different states below. Figure 3: Characterization of spin–photon entanglement. ( a ) The laser pulse sequence used for the generation of spin–photon entangled state and measurement of quantum correlations after a spin-echo sequence. ( b ) Spin–photon entanglement in the rotated basis and the relevant energy-level diagram (right inset). QD2 is prepared in the single-electron charged state and an external magnetic field of B x =0.7 T is applied in the Voigt geometry. The main figure shows the photon detection events as a function of time, during and after the entanglement generation pulse, conditioned upon a spin-echo-delayed spin measurement in the state. The entanglement generation pulse is turned on at time t =0 and is 1.2 ns long. The oscillations in the depicted coincidence counts at Δ= ω b – ω r =4.9 GHz are due to the beating between the two frequency components of the projected single-photon superposition state. The vertical dashed line indicates the entangled spin–photon generation time, for which the spin-echo sequence exactly cancels the random phase accumulated due to hyperfine interactions. The error bars represent 1 s.d., deduced from poissonian statistics of the raw detection events. Full size image For an echo time T echo =13 ns, a measurement of the spin–photon correlations in a rotated basis is shown in Fig. 3b . Combined with measurements that project the photon and the spin in different states (see Supplementary Note 4 for details) we can calculate the spin–photon entanglement fidelity to be F >0.63±0.02: this bound is limited by the detection jitter (64 ps). If the detector jitter were absent, we would obtain 0.71±0.02 (0.82±0.02) as the lower bound for entanglement fidelity with (without) spin-echo. We emphasize that despite the similarity with the single-photon pulse shape in Fig. 2a , Fig. 3b depicts the time dependence of the coincidence counts as a function of generation time of the entangled spin–photon pair, with t =0 denoting the rise time of the entanglement generation pulse (see the pulse sequence depicted in Fig. 3a ). Teleportation from a photonic qubit to a spin qubit The state of the coupled system consisting of two photons in modes A and B and the QD spin prior to the beam splitter is If the photons in modes A and B are indistinguishable in every aspect but their internal (frequency/colour) state, the only possibility for a simultaneous coincidence detection at the output of the HOM interferometer is to have the input two-photon state in (ref. 8 ). Therefore, detection of a coincidence projects the input photonic state (in modes A and B) to | ϕ S › (ref. 1 ). To verify heralded quantum teleportation, the photonic qubit that is coupled to the mode A is generated by the neutral QD3, whose exciton transition energy is nearly identical to that of the QD2 trion (see the spectrum in Supplementary Fig. S3 ). To ensure that ω b – ω r of QD3 matches the electron Zeeman energy of QD2, a separate magnetic field of 0.12 T is applied to QD3. Moreover, the electric fields applied separately to the QD2 and QD3 are adjusted such that their emission frequencies ( ω b and ω r ) are identical. We focus on photons emitted in an 800 ps long time-interval, slightly longer than the 650 ps QD lifetime (as depicted in Fig. 4a ), and observe coincidences at the outputs of the HOM interferometer at a rate of ~2 s −1 . The spin state corresponding to this measurement outcome is ‹ ϕ S |Ψ›= α |↑›+ β |↓›, as can be verified from equation (2). 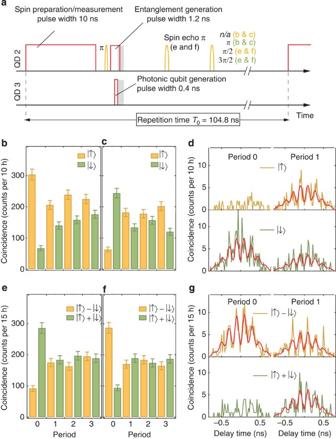Figure 4: Demonstration of quantum teleportation. (a) The experimental teleportation pulse sequence. The pulses applied to QD2 for entanglement generation are the same as inFig. 3. In the spin measurement stage, different combinations of spin rotation pulses are used. For QD3, 400 ps excitation pulses are used for generating the input photonic qubit. For teleportation, we use the coincidences at the two outputs of the HOM interferometer in an 800 ps long time-interval (labelled as the grey box). (b,c) Teleportation with input qubit |ωr› (b) or |ωb› (c). The plots show three-fold coincidence counts between the two output arms of the beam splitter and a photon detection during the following spin measurement pulse (Period=0) or during a later pulse period (Period>0). The green and yellow columns represent different spin measurement basis. An enhanced probability for the spin state |↑› (|↓›) as well as a decreased probability for |↓› (|↑›) is observed when the photonic qubit was initially prepared in |ωr› (|ωb›). The error bars represent 1 s.d., deduced from poissonian statistics of the raw detection events. (d) Time resolved three-fold coincidence counts in the first two periods inc. Red lines represent the expected two-photon interference oscillations (seeSupplementary Note 2). The delay time represents the difference in the photon detection time at the output of the HOM interferometer. (e,f) Same asbandcbut with different input qubit |ωr›+|ωb› (e) or |ωr›–|ωb› (f). A spin-echoπ-pulse is applied to prolong the spin coherence time. (g) Time-resolved coincidence counts in the first two periods inf. Figure 4: Demonstration of quantum teleportation. ( a ) The experimental teleportation pulse sequence. The pulses applied to QD2 for entanglement generation are the same as in Fig. 3 . In the spin measurement stage, different combinations of spin rotation pulses are used. For QD3, 400 ps excitation pulses are used for generating the input photonic qubit. For teleportation, we use the coincidences at the two outputs of the HOM interferometer in an 800 ps long time-interval (labelled as the grey box). ( b , c ) Teleportation with input qubit | ω r › ( b ) or | ω b › ( c ). The plots show three-fold coincidence counts between the two output arms of the beam splitter and a photon detection during the following spin measurement pulse (Period=0) or during a later pulse period (Period>0). The green and yellow columns represent different spin measurement basis. An enhanced probability for the spin state |↑› (|↓›) as well as a decreased probability for |↓› (|↑›) is observed when the photonic qubit was initially prepared in | ω r › (| ω b ›). The error bars represent 1 s.d., deduced from poissonian statistics of the raw detection events. ( d ) Time resolved three-fold coincidence counts in the first two periods in c . Red lines represent the expected two-photon interference oscillations (see Supplementary Note 2 ). The delay time represents the difference in the photon detection time at the output of the HOM interferometer. ( e , f ) Same as b and c but with different input qubit | ω r ›+| ω b › ( e ) or | ω r ›–| ω b › ( f ). A spin-echo π -pulse is applied to prolong the spin coherence time. ( g ) Time-resolved coincidence counts in the first two periods in f . Full size image Experimental verification of teleportation is based on three-fold coincidence detection of photons at the two output modes of the HOM interferometer, together with a photon detection during the spin-measuremement/preparation pulse. The spin population in the |↑› before the start of the spin-measuremement/preparation pulse determines the probability that resonantly excited QD scatters/emits one or more photons. After a few optical excitation/emission cycles, the spin is pumped to the |↓› state and the QD resonance fluorescence ceases. Owing to the modest collection efficiency of our set-up, a photon is detected with 0.3% probability if the initial population is in |↑›. We emphasize however that once a photon is detected, we can tell that the spin state immediately prior to the spin measurement pulse was in |↑› with a high confidence level. To detect the spin in other states we apply a carefully chosen rotation pulse prior to the spin measurement/preparation pulse; the rotation pulse coherently maps a desired spin state to |↑› state and thus allows us to identify if the spin prior to the rotation pulse was in the targeted spin state. In order to demonstrate classical correlations between the colour of the photon to be teleported and the final spin state, we use an input photon that is prepared either in or and measure the spin state projected to either |↑› or |↓›. For a mode A photon in | ω r › A , a three-fold coincidence projects the photon in mode B onto | ω b › B and the spin onto |↑›. Figure 4b shows that the same period (Period 0) three-fold coincidences corresponding to a spin measurement in |↑› are a factor ~4 larger than those corresponding to |↑›. By using an input photon in state | ω b › A , the three-fold coincidences in Period 0 show that detecting the spin in |↓› is now ~4.0 more likely than detecting it in |↑› ( Fig. 4c ), in accordance with the predictions of the teleportation protocol. From these measurements, we obtain the teleported state fidelities 0.79±0.1 (0.82±0.09) for | ω r › A (| ω b › A ), where the fidelity for each teleported state is calculated as the overlap of the ideal electron spin state after the completion of the protocol with the corresponding experimental outcome for the spin state (see Supplementary Note 6 for details). The different period three-fold coincidences are obtained by correlating the coincidence events for photons at the output of the HOM interferometer generated within the same period, with a spin measurement in the subsequent period. The corresponding coincidences, labelled as Period 1, also show a difference between the spin-up and spin-down populations, but this difference is due to a steady-state population difference between the two spin states and is not affected by the photonic qubit state (see Supplementary Note 6 for more information). Demonstration of quantum teleportation requires that coherences in the photonic superposition state at the input mode A are faithfully transferred onto the spin state. To verify this, we prepare the single photon in mode A in either | ω r › A +| ω b › A or | ω r › A −| ω b › A . As the propagation time of the photons onto the super-conducting-single-photon detector (SSPD) is about 11 ns, we introduce the spin-echo pulse sequence described in the previous section to ensure that the spin measurement is carried out only after the coincidence detection at the output of the HOM interferometer. The three-fold coincidences now indicate an enhanced probability for detection of the spin in state |↑›+|↓› for an input photon in | ω r › A +| ω b › A ( Fig. 4e ) and |↑›−|↓› for an input photon in | ω r › A −| ω b › A ( Fig. 4f ). From these measurements, we obtain the teleported state fidelities 0.76±0.03 (0.75±0.03) for | ω r › A +| ω b › A (| ω r › A –| ω b › A ). Slightly higher teleportation state fidelities 0.80±0.03 (0.78±0.03) have been achieved in the case without the spin-echo pulse sequence (see Supplementary Note 5 ). We remark that the time-resolved three-fold coincidence data shown in Fig. 4d,g exhibit beat notes that have a different origin from those appearing in Fig. 2a due to single-photon interference. The oscillations at frequency ω b – ω r =4.9 GHz in Fig. 4d stem from a two-photon interference between a photon at ω b and a second one at ω r as in ref. 39 (see Supplementary Note 2 ). We emphasize that unlike the case in Fig. 2b , the photons incident on the HOM interferometer are generated in the same excitation period even for the three-fold coincidences depicted in Period 1. As the spin detection takes place in the subsequent period, one of the photons incident on the HOM interferometer is effectively in a mixed state. The beat in the Period 1 therefore corresponds to the interference between the state | ω b › and the mixed state | ω b ›‹ ω b |+| ω r ›‹ ω r |, giving rise to an interference pattern that is identical to that obtained between | ω b › and | ω r › in Period 0. Similarly, the oscillations in Fig. 4g come from a two-photon interference between a photon at | ω r ›−| ω b › and the second one either at | ω r ›+| ω b › (Period 0) or a completely mixed state (Period 1) [39] . The measured teleported state fidelities are primarily limited by the small mismatch between the temporal pulse shapes and the spatial overlap profiles of the two interfering photons, as well as the finite spin–photon entanglement fidelity stemming from hyperfine interaction-mediated electron spin decoherence. We emphasize that, unlike measurements of entanglement fidelity [34] , [35] , [36] , the experimentally determined teleportation fidelity is independent of the detector jitter. Prolongation of the spin-echo time beyond 25 ns in our experiments is limited by dynamical nuclear spin polarization effects [40] , [41] that are omnipresent in self-assembled QDs (see Supplementary Note 3 ). The relatively short timescale in which teleportation can be observed for QD2 limits possible applications of teleportation where longer memory times are needed. We note that at higher magnetic fields spin T 2 coherence times exceeding 1 μs have been reported for single InAs QDs [40] : future work is needed to understand and extend the timescale that currently limits the memory time we observe. The three-fold coincidence rate in our experiment is about 19 h −1 . The two-fold coincidence rate of the interfering photons in the Bell basis measurement is about 1.7 s −1 . Defining D 3 ( D 2 ) as the detection efficiency of photons from QD3 (QD2) without the beam splitter, we estimate D 3 =0.15% and D 2 =0.05%. Furthermore, using the number of successful teleportation events, we estimate the spin detection efficiency to be D spin =0.30%. The difference between D 3 and D 2 is mainly due to the difference between the collection efficiency of the emitted photons from the two QDs and the different powers used for generating the photonic qubit and the entanglement state. We note here that D 2 is six times lower than D spin due to the fact that on average two photons are scattered during the spin measurement, and that we use a laser power that is less than what is needed for implementing a π pulse in the entanglement generation pulse. Finally, the 800 ps detection window also reduces the detection probability of a single photon that is entangled with the spin. The limitation in the count rate here is mainly caused by the photon extraction efficiency from the QD sample ( 10%), the loss in the collection system and the detection efficiency (35%). The teleportation protocol we implemented is probabilistic due to a 25% efficiency of the Bell state measurement corresponding to a coincidence detection in the HOM interferometer. In the current experiment, we demonstrate an average teleported state fidelity of 0.78±0.03 (0.80±0.03) with (and without) spin-echo sequences, for four states that lie on a plane on the Bloch sphere; for such states, the optimal state estimation yields a fidelity of 3/4 and our result is above this classical limit by 1 (1.67) standard deviation [42] . Universal quantum teleportation requires that the protocol is implemented for six photonic states that do not lie on a plane: in that case, an average teleportation fidelity exceeding 2/3 is required to demonstrate quantum teleportation [43] . As discussed in the previous section, the principal mechanisms that limit the measured fidelities are imperfect two-photon interference visibility, imperfect entanglement fidelity and hyperfine interaction induced spin decoherence. As these mechanisms lead to a similar reduction of fidelity for photonic states that are eigenstates of σ y or σ x , we would expect the corresponding teleported state fidelities to be comparable. We remark that extension of our experiments to demonstrate universal teleportation presents no difficulties as it is straightforward to generate the photonic qubit in an arbitrary superposition of | ω b › and | ω r › by placing the excitation and detection polarizers at other angles relative to the QD transitions and also by adjusting the relative phase φ L . For the spin state, the measurement in the different basis can be performed by changing the power and time delay of the spin rotation pulse. We expect quantum teleportation from a propagating photonic qubit to a stationary solid-state spin qubit to have a central role in quantum networks where nodes incorporating a small number of spin qubits are interconnected using photons. Although the finite efficiency of quantum state transfer is in general an important limitation, the heralding of successful transfer renders the implemented protocol relevant for schemes such as linear optics quantum computation which rely on post-selection on measurement results and where quantum memory for the photons is crucial. We note that the teleported state of the photon can be retrieved from the QD spin and transferred onto another photonic qubit using resonant excitation and further post-selection (see Supplementary Note 7 ), albeit with low efficiency. As our photonic qubit is generated by a neutral QD exciton, our experiment can also be considered as the realization of teleportation from the exciton qubit of one QD to the spin qubit of another QD. A natural extension of the quantum teleportation protocol is to entangle the spin states of two distant QDs that have never directly interacted with each other [44] , [45] . To entangle two spins one would replace the photonic qubit with a photon that is entangled with another QD spin: a coincidence detection at the output of the HOM interferometer, in this case, heralds successful generation of entanglement between the two distant spins. Further interesting extensions include quantum teleportation to a decoherence-avoiding singlet–triplet qubit in a QD molecule [46] , to a hole spin [47] , or a subsequent transfer of the spin state from the self-assembled QD to a gate-defined QD, where longer coherence times on the order of 200 μs and coherent two-qubit gates have been demonstrated [48] . Synchronization Two synchronized optical set-ups are used to excite the two QDs that create the photonic qubit and the spin–photon entangled pair (see Supplementary Fig. S1 ). For the generation of the spin–photon entangled pair, ns pulses used for resonant excitation of the QD are combined with ps pulses used for spin rotation. A mode-locked Ti:sapphire laser produces ps pulses at a rate of 76.3 MHz. An amplitude electro-optic modulator (A-EOM 1) is used as a pulse picker, decreasing the pulse rate to 9.5 MHz (104.8 ns repetition period). Pulses are divided and recombined using a series of beam splitters, and some are delayed by precise amounts of time using translation stages. We produce a sequence of three ps pulses used as spin rotation pulses, which are then combined with ns pulses produced from a continuous-wave Ti:sapphire laser by another EOM (A-EOM 2) that are used to resonantly excite QDs. In the second set-up, 400 ps pulses from a tunable diode laser are generated by the third EOM (A-EOM 3). A Ph-EOM is further used to create frequency sidebands on the laser, used for two-colour resonant excitation of the QD. The fixed repetition rate of the mode-locked Ti:sapphire laser, measured by a fast photo-detector (PD1) is used as a reference to synchronize the generated pulses and the measurement. A microwave band-pass filter (MW filter) centred around 2.4 GHz picks the 32nd harmonic of the reference signal, which is then amplified (MW ampl) and fed into the clock input of the pulse pattern generators (PPGs) 2 and 3. A 76 MHz signal generated from PD2 is used to synchronize the PPG1 driving the pulse picker EOM (A-EOM 1). Experimental set-up Two liquid helium bath cryostats operating at ~4 K, separated by ~5m, host the two QDs. In both cryostats, a fibre-coupled confocal microscope focuses the excitation laser pulses onto the QD using a high NA (0.6) objective. The QD emission is collected through the same objective and coupled into a collection fibre. Excitation laser background is suppressed by a polarizer that transmits the component of the emission that is orthogonally polarized with respect to the laser. Photons from the QDs are sent through diffraction gratings ( 70 GHz bandwidth) to eliminate the phonon sideband emission and are incident on a beam splitter where they interfere. The two output arms of the beam splitter are coupled to SSPDs with high quantum efficiency (35% at 960 nm) and low jitter (64 ps). A time-correlated single-photon counting module (TCSPC) is used to measure correlations between the photons on the two output arms of the beam splitter. In order to reduce the collected data, a 60 kHz time tagger generated by prescaling the 2.4 GHz reference signal, is used as the synchronization clock of the TCSPC. In the HOM interferometer set-up, both QDs are excited by the same laser. The photons from the QDs are combined on a beam splitter and the output modes are sent to two SSPDs, completing the HOM interferometer (see Supplementary Fig. S4 ). The path lengths of the two arms of the interferometer, between the first and the second beam splitter, are made identical to ensure a good temporal overlap of two photons. The polarization is adjusted using fibre paddles in the two arms of the interferometer. In the teleportation experiment, we use the same two detectors for detecting the interfering photons and the photons emitted during the spin measurement pulse, using their emission time to distinguish between them. The entanglement generation pulse and the spin measurement pulse are separated by 92 ns: this delay ensures that the photons emitted during the spin measurement pulse arrive at the detectors after the dead time (90 ns) of the TCSPC. How to cite this article: Gao, W. B. et al. Quantum teleportation from a propagating photon to a solid-state spin qubit. Nat. Commun. 4:2744 doi: 10.1038/ncomms3744 (2013).